A very long-term transient event preceding the 2011 Tohoku earthquake Geodetic transients have been observed in various subduction zones. The 2011 Tohoku earthquake occurred in one of the most active subduction zones globally, the Japan Trench subduction zone (JTSZ). However, no geodetic transient (except afterslip and so on) had been reported in the JTSZ before the Tohoku earthquake. Here we show that a large transient event, with duration longer than any reported previously, occurred in the JTSZ preceding the Tohoku earthquake. We calculate tectonic deformations at Global Positioning System stations along the JTSZ by removing the effects of nearby M w 6–8 earthquakes. We identify temporal changes in these deformations, deriving 9-year deviation records from regular deformations due to slip deficit at the plate boundary. We perform an inversion of the deviations to obtain the source model of their root event. The relationship between the obtained transient event and Tohoku earthquake is shown through Coulomb stress change and seismic supercycle simulation. Geodetic transients have been observed in various subduction zones [1] , [2] , [3] and have long been believed to be the key phenomena associated with megathrust earthquakes, although the nature of this relationship remains elusive [4] . Indeed, it has been reported that geodetic transients might have preceded megathrust earthquakes [5] . For example, long-term slow slip events (SSEs), which are those with duration longer than 10 7 s (ref. 3 ) were observed before the 1983 Japan Sea earthquake along the boundary of the Eurasian and North American plates [6] and before the 2012 Ometepec earthquake in the southern Mexico subduction zone [7] . However, in one of the most active subduction zones in the world, the Japan Trench subduction zone (JTSZ), where the 2011 Tohoku earthquake [8] , [9] occurred with a moment magnitude ( M w ) of 9.0, no geodetic transient had been reported previously; rather, only afterslip, short-term silent earthquakes and recovery of plate coupling had been reported [3] , [10] . In fact, even in the period immediately before the Tohoku earthquake, only short-term transients around the foreshock were reported [11] , [12] . Nevertheless, tectonic deformations due to drag of the overriding plate coupled with the subducting plate (slip deficit) were being observed continuously in the JTSZ, and any geodetic transients that occurred in the region should have affected these tectonic deformations. To investigate this phenomenon, we first analyse the temporal changes in tectonic deformations before the Tohoku earthquake. We use a data set from the dense Global Positioning System (GPS) network GEONET, operated by the Geospatial Information Authority of Japan (GSI). In previous studies [13] , [14] , [15] , [16] , the slip deficit rate in the JTSZ was imaged using partial data sets covering the period of seismic quiescence before the 2003 Tokachi-oki earthquake. In this study, we use the whole data set from 21 March 1996 to 8 March 2011 (one day before the foreshock). Time series of deformation We converted the daily coordinates of the GEONET stations in the Tohoku and Kanto districts along the JTSZ to time series of horizontal deformation (see Methods). Sinusoidal annual variations and the co-seismic and post-seismic signals of nearby M w 6–8 earthquakes are apparent in the results of this conversion ( Fig. 1a,b ). In addition, stationary westward trends were obtained at all stations for the seismic quiescence period before 2002 (red lines in Fig. 1b ), and we assumed that these represent regular deformations that were due to slip deficit, as in all previous studies [13] , [14] , [15] , [16] . We conducted an additional analysis of the time series; the results shown in Supplementary Note 1 and Supplementary Fig. 1 can also support our assumption. 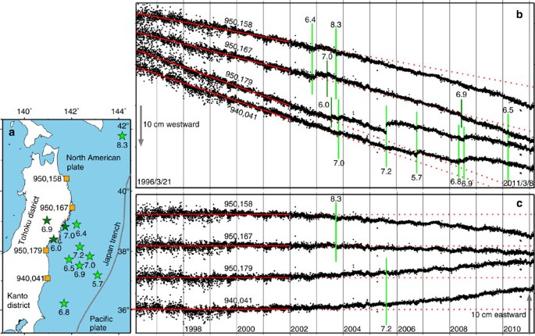Figure 1: Time series of east–west deformation at GPS stations in the Tohoku district. (a) Selected GPS stations (orange squares) andMw6–8 earthquakes (green stars) in the index map. (b) Original time series of east–west deformation obtained from the GEONET F3 solutions34at the stations and the effects of theMw6–8 earthquakes (green lines). (c) Detrended time series obtained by removing the regular trends in 1996–2001 (solid red lines), annual variations and earthquake effects. These time series deviated from the zero lines around 2002 and accelerated at the time of the 2003 or 2005 earthquake (green lines). Figure 1: Time series of east–west deformation at GPS stations in the Tohoku district. ( a ) Selected GPS stations (orange squares) and M w 6–8 earthquakes (green stars) in the index map. ( b ) Original time series of east–west deformation obtained from the GEONET F3 solutions [34] at the stations and the effects of the M w 6–8 earthquakes (green lines). ( c ) Detrended time series obtained by removing the regular trends in 1996–2001 (solid red lines), annual variations and earthquake effects. These time series deviated from the zero lines around 2002 and accelerated at the time of the 2003 or 2005 earthquake (green lines). Full size image We removed the annual variations and co-seismic and post-seismic signals from the time series by fitting trigonometric, Heaviside and logarithmic functions. Then, we performed regression analyses for the pre-2002 parts of the time series to determine the trends of regular slip deficit deformations and removed the obtained trends from the time series, as for the Tokai SSE [1] and Bungo Channel SSE [17] . If the slip deficit deformations were the only parameters affecting the results, the data should be distributed around the zero line. However, the obtained data began to deviate from the zero line around 2002 ( Fig. 1c ). This deviation was eastward at the central and southern stations, where movement was accelerated at the time of the 2005 M w 7.2 Miyagi-oki earthquake, but westward at the northern stations, where movement was accelerated at the time of the 2003 M w 8.3 Tokachi-oki earthquake (green lines in Fig. 1c ). The total deviations at all stations were measured from the vertical coordinates on 8 March 2011 in time series diagrams such as that illustrated in Fig. 1c . 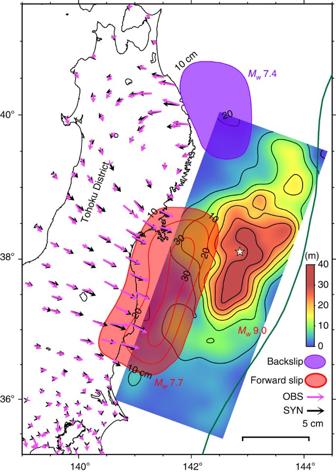Figure 2: Distribution of total deviations and the result of a two-source inversion. The red and purple contours represent the distributions of the forward slip by the very long-term transient event and the backslip by the northern source, which were obtained through the two-source inversion of the total deviations (pink arrows). The black arrows denote synthetic deviations computed for the inversion result. The co-seismic slip distribution of the 2011 Tohoku earthquake8is also displayed with the epicentre (white star) and Japan Trench (dark green line). The black bar at the bottom right denotes 100 km. Characteristics of the sources of deviations Figure 2 shows the distribution of measured total deviations (pink arrows). As found in deformation accelerations [18] and deformations including post-seismic signals [9] , [19] , [20] , large eastward deviations were observed along the eastern coast of central and southern Tohoku with a broad extension to the west. Meanwhile, westward deviations are obvious in the data obtained for northern Tohoku, although there was no significant deviation in the Kanto district. Small southward deviations were found extending along the western coast of northern Tohoku, as has been found previously in deformation accelerations [18] . This implies that the sources of the large eastward and westward deviations were located far from the western coast. Small southward deviations were also detected along the boundary between central and northern Tohoku, where the large eastward and westward deviations cancelled each other out. Figure 2: Distribution of total deviations and the result of a two-source inversion. The red and purple contours represent the distributions of the forward slip by the very long-term transient event and the backslip by the northern source, which were obtained through the two-source inversion of the total deviations (pink arrows). The black arrows denote synthetic deviations computed for the inversion result. The co-seismic slip distribution of the 2011 Tohoku earthquake [8] is also displayed with the epicentre (white star) and Japan Trench (dark green line). The black bar at the bottom right denotes 100 km. Full size image On the basis of the above-mentioned evidence, we assumed the two sources to be located on deeper parts of the plate boundary beneath and off the eastern coast of central and southern Tohoku or northern Tohoku. The northern source for the westward deviations was interpreted previously to be a result of recovery of plate coupling [10] or temporary acceleration of subduction [21] . These interpretations cannot be applied to the southern source, because this source generated deviations in the opposite direction. However, the deviation direction and source position relative to the Tohoku earthquake are similar to those of the Tokai SSE [1] relative to the 1854 M 8.4 Tokai earthquake and the Bungo Channel SSE [17] relative to the 1707 M 8.6 Hoei earthquake. The detrended time series at stations in central and southern Tohoku from during 2002 to August 2005 and from August 2005 to March 2011 are as stationary as those of the Tokai and Bungo Channel SSEs, as shown in Fig. 1c . A more similar case was found in the Alaska subduction zone, where long-term SSEs with duration of several years were observed downdip to the source region of the 1964 M 9.2 Alaska earthquake [22] . Therefore, we can consider the southern source to be a phenomenon like a long-term SSE, but this would have a total duration of about 9 years, longer than any long-term SSE reported previously; thus, we refer to it as a very long-term transient event, following the terminology in simulation studies [23] , [24] . In contrast to short-term SSEs, long-term SSEs and their relatives are not always accompanied by tremor activities, although, if an episodic tremor and slip (ETS) zone exists in the vicinity of a long-term SSE, the SSE can excite tremor activity in the ETS zone [4] . However, no ETS zones have been found in the JTSZ, and the very long-term transient event was not accompanied by tremor activities. Inversion of the deviations for finite source models Because deformation due to slip deficit is westward and slip deficit is traditionally modelled according to a normal faulting mechanism consisting of backslips [25] , [26] , the very long-term transient event for eastward deviations can be modelled according to a reverse faulting mechanism consisting of forward slips. Consequently, we located a dipping rectangular reverse fault on the deeper part of the plate boundary in central and southern Tohoku to explore the source characteristics of the very long-term transient event by analysing the deviations. However, we also had to introduce a dipping rectangular normal fault in northern Tohoku, because this northern backslip source affected deviations not only along but also beyond the boundary between northern and central Tohoku. Then, we performed an inversion of the deviations for finite source models of the very long-term transient event and northern backslip source (see Methods). The resultant slip distribution and M w of 7.7 are shown in Fig. 2 , accompanied by those for the northern backslip source ( M w 7.4) and previous results obtained for the Tohoku earthquake ( M w 9.0) (ref. 8 ). The synthetic deviations (black arrows in Fig. 2 ) indicate that southeastward deviations to the northwest of the very long-term transient event and southwestward deviations to the southwest of the northern backslip source resulted in the small southward deviations observed along the western coast of northern Tohoku. The forward slip distribution of the very long-term transient event is slightly different from that of a previous study [9] , because we excluded post-seismic deformations of nearby M w 6–8 earthquakes from the data, and constrained the location of the very long-term transient event to be similar to the relative locations of the Tokai and Bungo Channel SSEs as mentioned in the previous section. The lower two time series in Fig. 1b , which were observed at the stations in central and southern Tohoku, never became flat even after the very long-term transient event started. This means that, although the transient event was as large as M w 7.7, the rates of deformations caused by this event never exceeded those due to the slip deficit. However, this is quite typical for a large transient event because the average slip rate is expected to be 6.3 cm per year based on the M w and the scaling law of ν =10 9.5- Mw mm per year ( ν : slip rate) [27] . This value is only 74% of the actual subduction velocity, 8.5 cm per year. To examine the relationship between the very long-term transient event and the regular process consisting of the Tohoku earthquake and the slip deficit, we next computed changes in the Coulomb failure function (ΔCFF) [28] , as was conducted previously for the Tokai SSE [1] and simulated transient events [29] . The computations were performed for the focal mechanism and hypocentral depth of the Tohoku earthquake. A comparison of the ΔCFF distribution with the slip distribution of the Tohoku earthquake [8] in Fig. 3 indicates that the northern half zone of the large positive ΔCFF resulting from the very long-term transient event coincides with the main rupture area of the Tohoku earthquake, except for its trenchward extension. However, the northern backslip source distributed only negative or zero ΔCFF values throughout the rupture area of the Tohoku earthquake. Therefore, only the very long-term transient event affected the Tohoku earthquake. The ΔCFF values of the very long-term transient event, from near its upper edge to the hypocentre of the Tohoku earthquake, varied from +0.2 to +0.02 MPa, with an average of +0.1 MPa, around the mainshock hypocentre. This average is 20 times larger than the value found in the Tokai earthquake source area due to the Tokai SSE [1] , which did not lead to a megathrust earthquake. 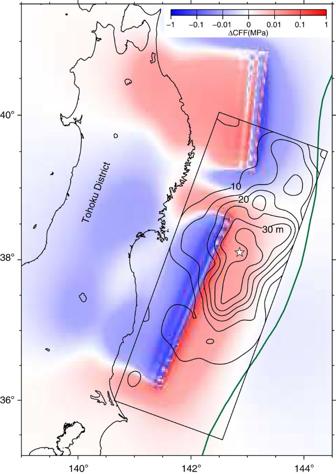Figure 3: Distribution of Coulomb failure function changes. The changes in the Coulomb failure function (ΔCFF)28, due to the very long-term transient event and northern backslip source, were computed for the focal mechanism and depth of the hypocentre (white star) of the 2011 Tohoku earthquake. The zones of positive and negative ΔCFF are indicated in red and blue, respectively. The co-seismic slip distribution of the 2011 Tohoku earthquake8and the Japan Trench are also displayed as black contours and the dark green line, respectively. Figure 3: Distribution of Coulomb failure function changes. The changes in the Coulomb failure function (ΔCFF) [28] , due to the very long-term transient event and northern backslip source, were computed for the focal mechanism and depth of the hypocentre (white star) of the 2011 Tohoku earthquake. The zones of positive and negative ΔCFF are indicated in red and blue, respectively. The co-seismic slip distribution of the 2011 Tohoku earthquake [8] and the Japan Trench are also displayed as black contours and the dark green line, respectively. Full size image Finally, we conducted a numerical simulation of megathrust earthquake cycles (seismic supercycles [30] ) to examine the possibility of a very long-term transient event in the JTSZ. We used the two-dimensional mechanical model [31] in Supplementary Fig. 2 and the method described in Methods. The velocity of the Pacific plate motion relative to the North American plate ( V pl ) is assumed to be 8.5 cm per year off central Tohoku, according to a plate kinematic model [32] . As in the original simulation [31] , the result of the simulation in Supplementary Fig. 3 indicates that a megathrust earthquake (large step) occurs every several hundred years, with large slips in the shallower regions around the Tohoku earthquake hypocentre (A, B and C) and smaller slips in the deeper region (D). Under such conditions, slip deficit accumulates (represented by long slopes) and M 7-class earthquakes (small steps in the slopes) occur during a supercycle between megathrust earthquakes. Moreover, several very long-term transient events (flat parts in the slopes) also occur in D during a supercycle, with the last one occurring just before and leading to a megathrust earthquake. In short, the interseismic period of a supercycle should consist primarily of three phenomena: the slip deficit of the regular process, M 7-class earthquakes and very long-term transient events. Therefore, the 2002 to March 2011 parts of the time series shown in Fig. 1b should represent the sum of the effects of these three phenomena. However, because the crustal and in-slab earthquakes (dark green stars in Fig. 1a ) do not belong to the category of M 7-class earthquake defined above, we removed their co-seismic and post-seismic signals (dark green lines in Fig. 1b ) from the time series. We measured composite deformations due to the three phenomena from the revised time series, as shown with pink arrows in Supplementary Fig. 4 . Then, we performed an inversion of the composite deformations for a source model extending along the Japan Trench, and computed ΔCFF values due to the resultant slip distribution (purple contours in Supplementary Fig. 4 ), finding the composite ΔCFF around the mainshock hypocentre to be ~+1 MPa. Considering the results of both the seismic supercycle simulation and the two ΔCFF computations, it is proven that a very long-term transient event occurred over the 9 years preceding the 2011 Tohoku earthquake. We also suggest that this transient event could have led to the advancement of the occurrence time [33] of the Tohoku earthquake, contributing 10% to the composite ΔCFF. The above simulation did not perfectly reproduce these findings; performing an extensive set of simulations with new inputs would provide further understanding of the physics governing such transient events and their relationship to a megathrust earthquake like Tohoku. Interseismic deformation The GSI is analysing GPS data from their GEONET using the Bernese GPS software (version 5.0), IGS ephemerides, and ITRF2005 (ref. 34 ). The results of the analyses are being published as the F3 solutions for the daily coordinates of the GEONET stations [34] . The F3 solutions for stations in the Tohoku and Kanto districts from 21 March 1996 to 8 March 2011 were adjusted by removing the motion of the North American plate in the plate kinematic model [32] . The adjusted coordinates were transformed into the Japan plane rectangular coordinate system VIII, IX or X (ref. 35 ). The horizontal components of deformation at each station were calculated from the obtained x - and y -coordinates. Source inversion scheme We performed the source inversion using a least-squares method with constraints [36] , although the positivity constraint on slip vectors was not applied because the observed deviations include the effects of the very long-term transient event and the northern backslip source; thus, we had to model reverse- and normal-faulting sources simultaneously. Smoothness constraints with digital Laplacians remained, and their weights were determined by minimizing Akaike’s Bayesian Information Criterion [37] . Green’s functions were computed using the average one-dimensional velocity structure in and off the Tohoku and Kanto districts and the propagator matrix method with dynamic-static separation [38] . Seismic supercycle simulation The simulation was conducted using a two-dimensional mechanical model [31] and the method for media under the rate- and state-dependent friction law [39] . The plate boundary shape in the original model was revised to fit to the actual shape in and off central Tohoku. We also modified the distributions of parameters in the rate- and state-dependent friction law ( a − b , L and σ n eff ) (ref. 39 ) along the plate boundary. The unstable zone of a – b ~0 was extended to a depth over 60 km and the effective normal stress σ n eff was decreased at depths deeper than 40 km ( Supplementary Fig. 2 ). Other minor changes in a – b , σ n eff and L were also applied as shown in Supplementary Fig. 2 . How to cite this article : Yokota, Y. and Koketsu, K. A very long-term transient event preceding the 2011 Tohoku earthquake. Nat. Commun. 6:5934 doi: 10.1038/ncomms6934 (2015).